slanDCs selectively accumulate in carcinoma-draining lymph nodes and marginate metastatic cells Dendritic cells (DCs) initiate adaptive immune responses to cancer cells by activating naive T lymphocytes. 6-sulfo LacNAc + DCs (slanDCs) represent a distinct population of circulating and tissue proinflammatory DCs, whose role in cancer immune surveillance is unknown. Herein, by screening a large set of clinical samples, we demonstrate accumulation of slanDCs in metastatic tumour-draining lymph nodes (M-TDLN) from carcinoma patients. Remarkably, slanDCs are absent at the primary carcinoma site, while their selective nodal recruitment follows the arrival of cancer cells to M-TDLN. slanDCs surround metastatic carcinoma deposits in close proximity to dead cells and efficiently phagocytose tumour cells. In colon carcinoma patients, the contingent of circulating slanDCs remains intact and competent in terms of IL-12p70 and tumour necrosis factor alpha production, induction of T-cell proliferation and migratory capacity to a set of chemokines produced in M-TDLN. We conclude that activated slanDCs represent previously unrecognized players of nodal immune responses to cancer cells. Dendritic cells (DCs) consist of a heterogeneous population of circulating and tissue leukocytes [1] , [2] capable of directing adaptive T-cell immune responses to cancer cells [3] . DCs promote protective immunity by capturing antigens at the primary tumour site, migrating to lymph nodes via lymphatic vessels, and ultimately presenting these tumour-derived antigens to nodal naive T cells [1] , [2] , [4] . Alternatively, antigens can enter the lymph, reach the nodal marginal sinus and therein be captured and processed by nodal resident antigen-presenting cells [5] . In a clinically apparent tumour mass, however, the spontaneous immune response regularly fails to achieve a complete elimination of cancer cells, with DCs losing their adjuvant function and, similar to many other immune and non-immune cells, acquiring a tumour-promoting programme that sustains tumour escape [4] , [6] , [7] , [8] . In human blood, DCs are classically divided into three major subtypes: CD303 + plasmacytoid DCs (pDCs) and two CD11c + myeloid DC (mDC) subsets, namely a major subset represented by CD1c + (BDCA1 + ) DCs and a discrete CD141 + (BDCA3 + )/CLEC9A + DC subset [9] , [10] . Recently, a distinct population of peripheral and tissue proinflammatory DCs has been designated as 6-sulfo LacNAc + DCs (‘slanDCs’) based on its selective expression of the 6-sulfo LacNAc (slan) residue on the P-selectin glycoprotein ligand 1 membrane molecule, also known as M-DC8 (ref. 11 ). Circulating slanDCs represent 0.6–2% of peripheral blood mononuclear cells (PBMC) and are phenotypically distinct from pDCs and mDCs. They are, in fact, CD11c + /C3aR + /CD45RA + /6-sulfo LacNAc + and also characterized by a marked expression of CD16, as well as a very low expression of CD14 (ref. 12 ). Functionally, slanDCs stand out for their remarkable capacity to produce tumour necrosis factor alpha (TNFα) and IL-12p70 upon stimulation with discrete toll-like receptor ligands [13] , [14] . In addition, they are potent inducers of primary antigen-specific T-cell responses in vitro [11] , and show a superior programming of Th1/Th17 cell polarization as compared with classical CD1c + DCs [14] . Furthermore, slanDCs induce in vitro tumour-specific cytotoxic T cells and strongly promote natural killer (NK) cell proliferation, NK cytotoxic activity and, in cooperation with neutrophils, NK-derived interferon-gamma (IFNγ) production [15] , [16] , [17] . However, since the identification and functional analysis of human slanDCs in cancer patients has not been explored yet, in this study, we investigated such an issue. As a result, we uncover slanDCs as previously unidentified antigen-presenting cells that selectively accumulate in metastatic tumour-draining lymph nodes (M-TDLN) from carcinoma patients, where they likely participate in the organization of the nodal immune response. slanDCs populate the mucosal-associated lymphoid tissues In preliminary experiments, we comprehensively characterized the systemic distribution of human slanDCs under homoeostatic conditions. Human slanDCs can be specifically identified and monitored in formalin-fixed paraffin-embedded (FFPE) tissue sections by staining with DD2 and DD1 mAbs [17] that, similarly to the M-DC8 mAbs, recognize slan/M-DC8 (ref. 11 ). Tissue slanDCs were originally identified as M-DC8 + cells in the T-cell area of human tonsils by immunohistochemistry of frozen samples [18] . By using either DD2 or DD1, we confirmed that slanDCs are regularly found in nasopharyngeal (5/5 of our cases) and palatine (20/20 of our cases) tonsils, being particularly abundant in the crypts, where they strictly intermingle with epithelial cells ( Fig. 1a ). No reactivity in tonsils was detected by using isotype control antibodies ( Supplementary Fig. S1a,b ). More rarely, slanDCs were also found in the interfollicular area, whereas no DD2 + cells were found in the surface epithelium ( Supplementary Fig. S1c,d ). At high power view ( Fig. 1b ), the morphology of tonsil slanDCs appear heterogeneous, encompassing a dominant fraction of large cells with stellate morphology admixed to a minor cellular fraction of smaller cells with round-to-oval shape. In addition, most slanDCs were non-proliferating based on Ki-67 expression ( Supplementary Fig. S1e,f ). By analysing single-cell suspensions from human reactive tonsils, using a flow cytometry strategy recently reported [19] , we could confirm that among the various HLA-DR + /CD11c + DCs, slanDCs are clearly distinct from CD1c + (BDCA1 + ) DCs, CD141 + (BDCA3 + )/CLEC9A + DCs and CD14 high macrophages ( Fig. 1c–e ). 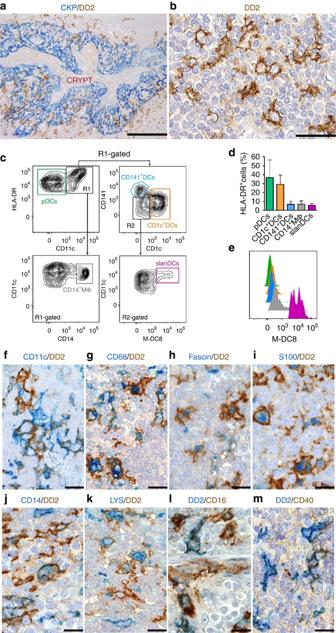Figure 1: Distribution and phenotype of slanDCs in human tonsils. Sections are from representative FFPE human tonsils and are stained as indicated by labels (CKP, pan-cytokeratin; LYS, lysozyme). (a) DD2+slanDCs surround the CKP+epithelium of tonsil crypts and mostly appear as large and stellate cells (b) (n=10). (c) Flow cytometry analysis was performed on live CD45+/HLA-DR+-singlet cells from CD3+/CD19+- depleted tonsil cell suspensions. The panel shows the gating strategy used to identify CD141+DCs (blue gate), CD1c+DCs (orange gate), CD14highMΦ (grey gate) and slanDCs (purple gate), within the HLA-DR+/CD11c+cells. By the same strategy, pDCs were identified within the HLA-DR+/CD11c−cells (green gate). A representative experiment out of three ones performed with similar results is shown. (d) Bar graph shows the percentage of each DC subset and macrophages within the HLA-DR+cells (mean±s.d.;n=5). (e) The histogram shows the relative expression of M-DC8 by each DC and MΦ populations. Data are representative of similar results obtained from five tonsil preparations. (f–m) Panels show representative DD2+slanDCs co-stained with antibodies towards a set of markers (n=10), as labeled. Sections are counterstained with Meyer’s haematoxylin. Original magnifications: 40X (a, scale bar, 500 μm); 400X (b,f–m, scale bar, 50 μm). Figure 1: Distribution and phenotype of slanDCs in human tonsils. Sections are from representative FFPE human tonsils and are stained as indicated by labels (CKP, pan-cytokeratin; LYS, lysozyme). ( a ) DD2 + slanDCs surround the CKP + epithelium of tonsil crypts and mostly appear as large and stellate cells ( b ) ( n =10). ( c ) Flow cytometry analysis was performed on live CD45 + /HLA-DR + -singlet cells from CD3 + /CD19 + - depleted tonsil cell suspensions. The panel shows the gating strategy used to identify CD141 + DCs (blue gate), CD1c + DCs (orange gate), CD14 high MΦ (grey gate) and slanDCs (purple gate), within the HLA-DR + /CD11c + cells. By the same strategy, pDCs were identified within the HLA-DR + /CD11c − cells (green gate). A representative experiment out of three ones performed with similar results is shown. ( d ) Bar graph shows the percentage of each DC subset and macrophages within the HLA-DR + cells (mean±s.d. ; n =5). ( e ) The histogram shows the relative expression of M-DC8 by each DC and MΦ populations. Data are representative of similar results obtained from five tonsil preparations. ( f – m ) Panels show representative DD2 + slanDCs co-stained with antibodies towards a set of markers ( n =10), as labeled. Sections are counterstained with Meyer’s haematoxylin. Original magnifications: 40X ( a , scale bar, 500 μm); 400X ( b , f – m , scale bar, 50 μm). Full size image By using an extensive panel of markers recognizing other tissue DCs and macrophages on FFPE sections, we found (either by immunohistochemistry or immunofluorescence) that a significant fraction of tonsil slanDCs co-express CD11c and CD68 (by using either KP1 or PG-M1 mAbs), and less frequently Fascin, nuclear S100 protein, CD14, lysozyme (LYS), CD16, CD40, myeloperoxidase, neutrophil elastase and factor XIIIa ( Fig. 1f–m and Supplementary Fig. S2 ), but are largely negative for markers restricted to pDCs (such as CD303 and CD123), Langerhans cells (such as CD1a and CD207), mature DCs (such as CD83 and CD208) and macrophages (such as CD163, CD11b and CD169). Positivity for a number of tonsil slanDC markers, including membrane M-DC8, were substantially confirmed on cytospin preparations of slanDCs purified from peripheral blood ( Fig. 2a–f ). On the other hand, flow cytometry studies of tonsil cell suspensions confirmed the lack of CD11b expression by tonsil slanDCs as opposed to the circulating counterpart [11] , suggesting that slanDCs downregulate CD11b once migrated into inflamed tonsils/tissues. 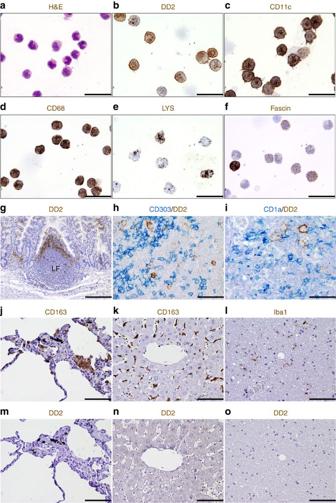Figure 2: Phenotype of slanDCs in peripheral blood and human tissues. (a–f) Panels are from cytospin preparations of freshly purified peripheral blood slanDCs, stained as labelled (LYS, lysozyme). Positivity is observed for all markers tested (n=5). (g–o) Sections are from human small bowel (g), reactive lymph node (h,i), normal lung (j,m), liver (k,n) and brain (l,o), and stained as labelled. M-DC8+slanDCs are numerous in Peyer’s patches (g), while in reactive lymph nodes CD303+pDCs (h) and CD1a+iDCs (i) are negative for M-DC8. On serial sections, CD163+alveolar macrophages (j,m), CD163+Kupffer cells (k,n) and Iba1+microglia (l,o) do not co-express M-DC8 (by DD2 staining). Sections are counterstained with Meyer’s haematoxylin. LF, lymphoid follicle. Magnification: 600X (a–f; scale bar, 33 μm), 100 × (g; scale bar, 200 μm), 400X (h,i; scale bar, 50 μm) and 200X (j–o; scale bar, 100 μm). Figure 2: Phenotype of slanDCs in peripheral blood and human tissues. ( a – f ) Panels are from cytospin preparations of freshly purified peripheral blood slanDCs, stained as labelled (LYS, lysozyme). Positivity is observed for all markers tested ( n =5). ( g – o ) Sections are from human small bowel ( g ), reactive lymph node ( h , i ), normal lung ( j , m ), liver ( k , n ) and brain ( l , o ), and stained as labelled. M-DC8 + slanDCs are numerous in Peyer’s patches ( g ), while in reactive lymph nodes CD303 + pDCs ( h ) and CD1a + iDCs ( i ) are negative for M-DC8. On serial sections, CD163 + alveolar macrophages ( j , m ), CD163 + Kupffer cells ( k , n ) and Iba1 + microglia ( l , o ) do not co-express M-DC8 (by DD2 staining). Sections are counterstained with Meyer’s haematoxylin. LF, lymphoid follicle. Magnification: 600X ( a – f ; scale bar, 33 μm), 100 × ( g ; scale bar, 200 μm), 400X ( h , i ; scale bar, 50 μm) and 200X ( j – o ; scale bar, 100 μm). Full size image DD2 or DD1 mAbs, on sections, also recognized slanDCs in the dome region of Peyer’s patches ( Fig. 2g ), but failed to identify sizeable numbers of slanDCs in other lymphoid organs such as the spleen, thymus and bone marrow. In most of the lymph nodes showing histology of nonspecific lymphadenitis (10/12 of cases), slanDCs were very rare with the exception of two cases characterized by a prominent follicular hyperplasia, in which we could detect CD68 + /CD11c + /DD2 + slanDCs in the extra-follicular area surrounding high endothelial venules (HEV). We also confirmed that DD2 does not recognize nodal CD303 + pDCs and CD1a + S100 + interdigitating DCs (iDCs), as indicated by double immunohistochemistry of sections from different forms of pDC- and iDC-rich lymphadenitis ( Fig. 2h,i ). Finally, Langerhans cells, interstitial DC (for example, dermal DCs), as well as different forms of specialized macrophages (for example, CD163 + alveolar macrophages, CD163 + Kupffer cells as well as Iba1 + microglia) were neither recognized by DD2 nor by DD1 mAbs ( Fig. 2j–o ). Altogether, these data confirm that DD2 and DD1 mAbs specifically and uniquely recognize tissue slanDCs in FFPE [13] , and establish that they are particularly abundant at the lymphoid–epithelial interface of mucosal-associated lymphoid tissues. slanDCs accumulate in M-TDLN of carcinoma patients slanDCs are known to accumulate in peripheral tissues during chronic and autoimmune inflammatory disorders, such as Crohn’s disease, rheumatoid arthritis and psoriasis [13] , [14] , [17] . Given their potent proinflammatory properties and propensity to tightly interact with epithelial cells, we posited that slanDCs could represent a hitherto unrecognized cellular component of the carcinoma microenvironment. To test this hypothesis, we used immunohistochemistry for M-DC8, as this marker is stable in slanDCs and apparently not inducible by tumour-cell-conditioned media in other monocyte/DC populations ( Supplementary Fig. S3 ). We initially screened reactivity for DD2 and DD1 clones on three distinct multi-tumour tissue microarrays (TMA) containing a total of 126 primary carcinomas (PCs) from different organs ( Supplementary Table S1 ). As expected, the large majority of the samples in the TMA showed infiltration by tumour-associated macrophages and DCs, as confirmed by stains for CD68 (100% of the cases), CD11c (99.2%), CD163 (the marker for M2-polarized macrophages, 99.2%) and CD1a (49.6%) ( Fig. 3a and Supplementary Fig. S4 ). In contrast, DD2 + /DD1 + slanDCs were rarely found (1.7%) ( Fig. 3a and Supplementary Fig. S4 ). 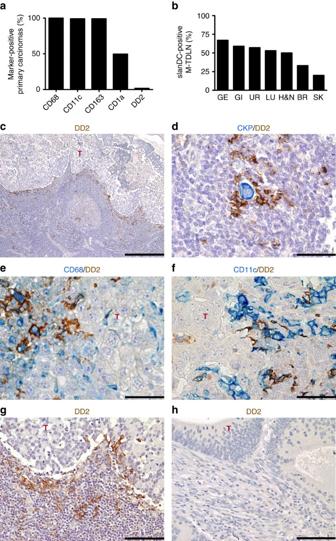Figure 3: Tumour-associated slanDCs are detectable only in M-TDLN. (a) Graph shows the frequency of carcinoma cases containing DC subsets and macrophages. Data have been obtained by scoring multi-tumour TMA sections stained for CD68, CD11c, CD163, CD1a and DD2 (n=3). (b) Graph shows the frequency of M-TDLN cases from different primary tumours containing slanDCs (GE, genital; GI, gastrointestinal; UR, urinary; LU, lung; H&N, head and neck; BR, breast; SK, skin). Data have been obtained by analysing a cohort of eighty M-TDLN on sections stained for DD2. (c–h) Sections are from M-TDLN stained as indicated. In M-TDLN, numerous slanDCs commonly line the nodal metastasis (c), while in cases with low tumour burden (d) slanDCs are found in close contact with dispersed single tumour cells. Double immunohistochemistry illustrates co-expression of CD68 (e) and CD11c (f) by DD2+slanDCs. (g,h) Comparative analysis of a slanDC-rich M-TDLN (g) with its matched primary carcinoma (h), the latter completely devoid of slanDCs in the surrounding tumour stroma. Sections are counterstained with Meyer’s haematoxylin. Original magnifications: 40X (c, scale bar, 500 μm); 600X (d–f, scale bar, 33 μm); 100X (g,h, scale bar, 200 micron). T, tumour cells. Figure 3: Tumour-associated slanDCs are detectable only in M-TDLN. ( a ) Graph shows the frequency of carcinoma cases containing DC subsets and macrophages. Data have been obtained by scoring multi-tumour TMA sections stained for CD68, CD11c, CD163, CD1a and DD2 ( n =3). ( b ) Graph shows the frequency of M-TDLN cases from different primary tumours containing slanDCs (GE, genital; GI, gastrointestinal; UR, urinary; LU, lung; H&N, head and neck; BR, breast; SK, skin). Data have been obtained by analysing a cohort of eighty M-TDLN on sections stained for DD2. ( c – h ) Sections are from M-TDLN stained as indicated. In M-TDLN, numerous slanDCs commonly line the nodal metastasis ( c ), while in cases with low tumour burden ( d ) slanDCs are found in close contact with dispersed single tumour cells. Double immunohistochemistry illustrates co-expression of CD68 ( e ) and CD11c ( f ) by DD2 + slanDCs. ( g , h ) Comparative analysis of a slanDC-rich M-TDLN ( g ) with its matched primary carcinoma ( h ), the latter completely devoid of slanDCs in the surrounding tumour stroma. Sections are counterstained with Meyer’s haematoxylin. Original magnifications: 40X ( c , scale bar, 500 μm); 600X ( d – f , scale bar, 33 μm); 100X ( g , h , scale bar, 200 micron). T, tumour cells. Full size image Given the low occurrence of slanDCs within PC, we then extended our analysis to metastatic tumour-draining lymph nodes (M-TDLN). Strikingly, slanDCs were numerous and easily detectable in 36/80 (45% of the cases) M-TDLN from carcinoma patients, whereas in the remaining 44/80 (55% of the cases), slanDCs were very rare or undetectable ( Supplementary Table S2 ). By cell counting, the density of slanDCs in M-TDLN was 283±96 mm 2 ( n =17). Of note, slanDCs were very rare or undetectable in all 155 non-metastatic TDLN draining breast carcinoma ( n =82), head and neck squamous cell carcinoma ( n =30), colon carcinoma ( n =28) and cutaneous melanoma ( n =15) ( Fig. 4a–d ). When the cohort of M-TDLN was segregated based on the site of origin of the PC, slanDC accumulation was found to be particularly frequent in M-TDLN draining carcinomas from the genital (67% of the cases), gastrointestinal (59% of the cases) and urinary tract (57% of the cases) ( Figs 3b and 4e–n,q,r ). The occurrence of slanDCs did not correlate with a specific subtype of the PC ( Supplementary Table S2 ). Notably, slanDCs were selectively located on the perimeter of metastatic nests within most M-TDLN, but only rarely infiltrated the tumour nests themselves ( Figs 3c , and 4e–h,m,n ). Even among M-TDLN cases containing rare slanDCs, the latter were selectively localized in close proximity to carcinoma cells, implying a tropism for transformed epithelial cells ( Fig. 3d ). Similar to slanDCs found in tonsils ( Fig. 1f,g ), slanDCs within M-TDLN co-stained for CD68 and CD11c ( Fig. 3e,f ) and were non-proliferating based on the lack of Ki-67 reactivity ( Supplementary Fig. S1g,h ). 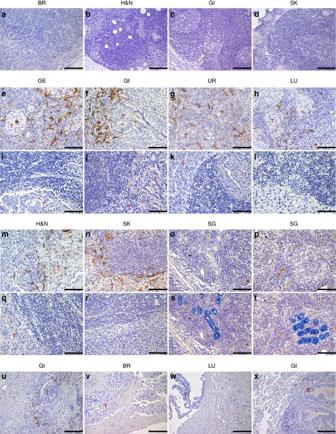Figure 4: slanDCs in human TDLN and carcinoma distant metastasis. Sections are from representative NM-TDLN (a–d;n=155) and M-TDLN (e–n,q–r;n=80), stained using the DD2 clone. slanDCs are virtually undetectable in NM-TDLN draining breast carcinoma (a), head and neck squamous cell carcinoma (b), colon carcinoma (c) and cutaneous melanoma (d). Examples of M-TDLN draining different primary sites including genital (GE;e,i), gastrointestinal (GI;f,j), urinary (UR;g,k), lung (LU;h,l), head and neck (H&N;m,q) and skin (SK;n,r), with (e–handm,n) or without (i–landq,r) slanDCs. (o,p,s,t) Sections are from salivary glands (SG)-draining LNs containing CKP+(blue) benign epithelial inclusions and co-stained for M-DC8 (brown); DD2 reactivity is limited to HEV. (u–x) Sections are from a set of representative carcinoma metastases (n=52) from different primary sites (indicate by labels) to the liver (u), brain (v), pleura (w) and lung (x); M-DC8+slanDCs are detectable only in a case with dense leukocyte infiltration (u). T, tumour cells. Sections were counterstained with Meyer’s haematoxylin. Original magnifications: 100X (a–d,u–x; scale bar, 200 μm) and 200X (e–t; scale bar, 100 μm). Figure 4: slanDCs in human TDLN and carcinoma distant metastasis. Sections are from representative NM-TDLN ( a – d ; n =155) and M-TDLN ( e – n , q – r ; n =80), stained using the DD2 clone. slanDCs are virtually undetectable in NM-TDLN draining breast carcinoma ( a ), head and neck squamous cell carcinoma ( b ), colon carcinoma ( c ) and cutaneous melanoma ( d ). Examples of M-TDLN draining different primary sites including genital (GE; e , i ), gastrointestinal (GI; f , j ), urinary (UR; g , k ), lung (LU; h , l ), head and neck (H&N; m , q ) and skin (SK; n , r ), with ( e – h and m , n ) or without ( i – l and q , r ) slanDCs. ( o , p , s , t ) Sections are from salivary glands (SG)-draining LNs containing CKP + (blue) benign epithelial inclusions and co-stained for M-DC8 (brown); DD2 reactivity is limited to HEV. ( u – x ) Sections are from a set of representative carcinoma metastases ( n =52) from different primary sites (indicate by labels) to the liver ( u ), brain ( v ), pleura ( w ) and lung ( x ); M-DC8 + slanDCs are detectable only in a case with dense leukocyte infiltration ( u ). T, tumour cells. Sections were counterstained with Meyer’s haematoxylin. Original magnifications: 100X ( a – d , u – x ; scale bar, 200 μm) and 200X ( e – t ; scale bar, 100 μm). Full size image Benign epithelial inclusions can be found in lymph nodes draining multiple body sites [20] , [21] . We asked if slanDC presence in LNs was specific to M-TDLN or whether slanDCs were normally present in LNs containing epithelial cells, even in the absence of malignancy. To this end, 13 non-inflamed, salivary gland DLN containing benign epithelial inclusions were examined, and 12/13 were found to be devoid of slanDCs ( Fig. 4o,p,s,t ), suggesting that nodal inflammation is required for slanDCs to gain access to the lymph node parenchyma. To further confirm the selective nodal tropism of slanDCs in carcinoma patients, multiple tissue blocks obtained from matched PC were analysed in a subgroup of 14 M-TDLN highly enriched in slanDC content. Expectedly, although the PC contained high numbers of tumour-associated DCs and macrophages, as proved by CD68, CD163, CD303, CD11c and CD1a staining, the large majority of them (12/14, 86.8%) were completely devoid of slanDCs, as shown by the comparative analysis of slanDC-rich M-TDLN with matched PC ( Fig. 3g,h ). Finally, slanDC infiltration was detected only infrequently in carcinoma distal metastases (3/52; 5.7% of the cases) ( Fig. 4u–x ). Collectively, these data suggest that slanDCs represent a new subset of distinct tumour-associated immune cells that are selectively recruited to M-TDLN. M-TDLN slanDCs are distinct from other M-TDLN DCs The distribution of slanDCs in M-TDLN was then compared with that of other canonical lymph node-resident DCs, namely pDCs and iDCs. In fact, within reactive human lymph nodes, including M-TDLN, CD303 + pDCs are selectively found in the extranodular compartment surrounding HEV [22] , [23] , whereas iDCs represent Langerhans-derived DCs, identifiable by the expression of CD1a, S100 protein and CD207 in the expanded paracortex of dermatopathic lymphadenitis [24] . In the 14 cases of slanDC-rich M-TDLN that we could test, CD303 + pDCs and CD1a + iDCs were expanded in their respective compartments ( Fig. 5a,b ). In addition, CD1a + DCs were also found within the tumour nests, whereas pDCs occasionally surrounded the nodal metastasis ( Fig. 5a,b ). In striking contrast, slanDCs were selectively found at the expansion front of the nodal metastatic deposit ( Figs 5c and 4e–h,m,n ), almost exclusively in contact with carcinoma cells. When tested by double immunohistochemistry, we found that both slanDCs and pDCs in M-TDLN were negative for CD83 and CD208/DC-LAMP ( Fig. 5d,e and Supplementary Fig. S5a,b ), consistent with a mostly immature phenotype, whereas a fraction of CD1a + iDCs were co-stained with both maturation markers ( Fig. 5f and Supplementary Fig. S5c ). On the other hand, slanDCs stained positive for HLA class II and CD40 molecules ( Fig. 5g,h ). In addition, a fraction of M-TDLN slanDCs (37±8%, n =4) also co-stained for cytoplasmic TNFα ( Fig. 5i ). This set of data suggests that slanDCs behave differently compared with other nodal DCs, as once recruited into the M-TDLN, they are partially activated and selectively localize adjacent to cancer cells. 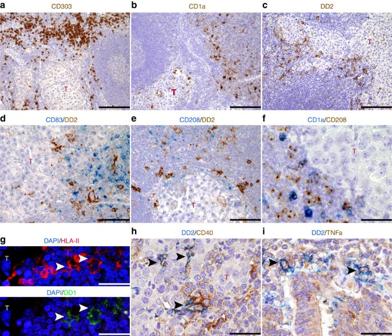Figure 5: Comparative analysis of tumour-associated DCs in M-TDLN. (a–i) Sections are from M-TDLN and stained as indicated. In this representative case (n=5), CD303+pDCs (a) and CD1a+iDCs (b) are mostly expanded in their own nodal compartments, with iDCs also infiltrating the tumour (T) nests, whereas DD2+slanDCs are found at the periphery of the tumour nodule (c). As shown by double staining, slanDCs are negative for CD83 (d) and CD208/DC-LAMP (e), at variance with CD1a+iDCs (f), but co-express HLA-II molecule (g), CD40 (h) and TNFα (i). Sections are counterstained with Meyer’s haematoxylin (a–fandh,i) and DAPI (g). Original magnifications: 100X (a–c, scale bar, 200 μm); 200X (d,e, scale bar, 100 μm); 400X (f, scale bar, 50 μm); 600X (g–i, scale bar, 33 μm). Figure 5: Comparative analysis of tumour-associated DCs in M-TDLN. ( a – i ) Sections are from M-TDLN and stained as indicated. In this representative case ( n =5), CD303 + pDCs ( a ) and CD1a + iDCs ( b ) are mostly expanded in their own nodal compartments, with iDCs also infiltrating the tumour (T) nests, whereas DD2 + slanDCs are found at the periphery of the tumour nodule ( c ). As shown by double staining, slanDCs are negative for CD83 ( d ) and CD208/DC-LAMP ( e ), at variance with CD1a + iDCs ( f ), but co-express HLA-II molecule ( g ), CD40 ( h ) and TNFα ( i ). Sections are counterstained with Meyer’s haematoxylin ( a – f and h , i ) and DAPI ( g ). Original magnifications: 100X ( a – c , scale bar, 200 μm); 200X ( d , e , scale bar, 100 μm); 400X ( f , scale bar, 50 μm); 600X ( g – i , scale bar, 33 μm). Full size image slanDC accumulation in TDLN represents an early event Subsequently, we took advantage of the sentinel lymph node (SLN) procedure to correlate slanDC nodal infiltration with the occurrence and progression of cancer cell colonization in TDLN. SLN biopsy is based on the assumption that cancer cells from a PC reach the SLN first, which can be accurately identified and then removed. In breast cancer, SLN biopsy represents a standard of care for nodal staging and might indicate a complete axillary lymph node dissection (ALND). Thus, for our analysis, we used 51 metastatic SLN (M-SLN) samples from patients with breast carcinoma. The presence of slanDCs in this cohort was documented in 17/51M-SLN (33.3% of the cases) ( Fig. 6a ), a similar frequency to what was observed in non-sentinel M-TDLN draining breast cancer (NSLN, 33.3% of the cases) ( Fig. 6a ). We then verified whether slanDC accumulation anticipates nodal metastasis and prepares tumour cell niches [25] . To this end, we analysed a subgroup of 22 cases of non-metastatic SLN (NM-SLN) and, remarkably, we found that only one NM-SLN case (1/22 (4.5%)) already contained slanDCs ( Fig. 6a ). Finally, we tested whether the presence of slanDCs in M-SLN could predict the ALND status in term of cancer cell colonization. We found that slanDC occurrence in M-SLN was not significantly associated with the ALND status (11/33 (33.3%) for tumour-negative ALND versus 4/18 (22.2%) for tumour-positive ALND, P =0.75) ( Fig. 6b–f ). Taken together, data suggest that, at least in human breast cancer, slanDC nodal accumulation in TDLN, although representing an early event (for example, colonization of the SLN), it is strictly coupled to nodal cancer cell colonization and cannot predict cancer dissemination to other nodes. 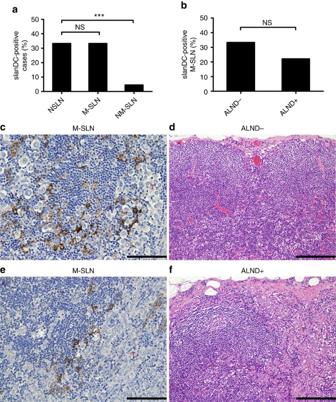Figure 6: slanDCs in breast cancer TDLN. (a) Graph illustrates the frequency of slanDCs in non-sentinel M-TDLN from the entire cohort (NSLN;n=80), metastatic breast cancer SLN (M-SLN;n=51) and non-metastatic breast cancer SLN (NM-SLN;n=22). (b) Graph illustrates the frequency of slanDCs in M-SLN with (ALND+) or without (ALND−) metastasis in the ALND (***P<0.0001;P>0.05 is nonsignificant (NS) by Fisher’s test). (c–f) Sections are from a representative M-SLN and matched ALND as indicated, and stained for DD2 (c,e) and H&E (d,f). T, tumour. Sections are counterstained with Meyer’s haematoxylin (c,e). Original magnifications: 200X (c,e, scale bar,100 μm) and 100X (d,f, scale bar, 200 μm). Figure 6: slanDCs in breast cancer TDLN. ( a ) Graph illustrates the frequency of slanDCs in non-sentinel M-TDLN from the entire cohort (NSLN; n =80), metastatic breast cancer SLN (M-SLN; n =51) and non-metastatic breast cancer SLN (NM-SLN; n =22). ( b ) Graph illustrates the frequency of slanDCs in M-SLN with (ALND + ) or without (ALND − ) metastasis in the ALND (*** P <0.0001; P >0.05 is nonsignificant (NS) by Fisher’s test). ( c – f ) Sections are from a representative M-SLN and matched ALND as indicated, and stained for DD2 ( c , e ) and H&E ( d , f ). T, tumour. Sections are counterstained with Meyer’s haematoxylin ( c , e ). Original magnifications: 200X ( c , e , scale bar,100 μm) and 100X ( d , f , scale bar, 200 μm). Full size image slanDCs are distinct from Tie2-expressing monocytes Our findings indicate that slanDCs are distinct from other tumour-associated DCs and macrophages in terms of distribution and location within the cancerous tissues. slanDCs are known to partially overlap [12] with the heterogeneous population of the CD16 + monocytes among PBMC (plots illustrating the gating strategy to identify the non-classical (CD14 dim /CD16 + ), intermediate (CD14 + /CD16 + ) and classical (CD14 + /CD16 − ) monocyte subsets, as well as slanDCs within the CD14 dim /CD16 + monocytes are displayed in Fig. 7a ) that have been also shown to include the Tie2-expressing monocytes (known as TEMs) [26] . The latter cells generate a perivascular cell population endowed with a prominent pro-angiogenic potential in a variety of human and mouse primary tumours, including human carcinomas [26] , [27] . However, even though circulating slanDCs, similarly to TEMs [26] , stain positively for CD16, CD33, CD13, CD11b and CD11c, but negatively for CCR2 and CD62L (ref. 11 ), they are distinct from TEMs as demonstrated by multiple evidence. First, circulating slanDCs are negative for Tie2 expression, unlike the CD14 + /CD16 + monocytes [28] , [29] as revealed by flow cytometry (using two different anti-Tie2 mAbs) ( Fig. 7b,c ). Second, lack of Tie2 expression by slanDCs was also confirmed by quantitative polymerase chain reaction ( Supplementary Fig. S6a ), and immunoblotting analysis (using two additional anti-Tie2 mAbs) ( Supplementary Fig. S6b ). Third, Tie2 mAbs failed to recognize any cells in the crypts of slanDC-rich tonsillar sections, where instead they stained only endothelial cells ( Fig. 7d ). Fourth, tumour-associated slanDCs are not perivascular and are only found in M-TDLN and not in PC, at variance with known patterns of TEM localization [26] . Finally, tumour-associated slanDCs do not express Tie2, as proven by immunohistochemical staining using an anti-Tie2 mAb suitable for FFPE tissues ( Fig. 7e ). 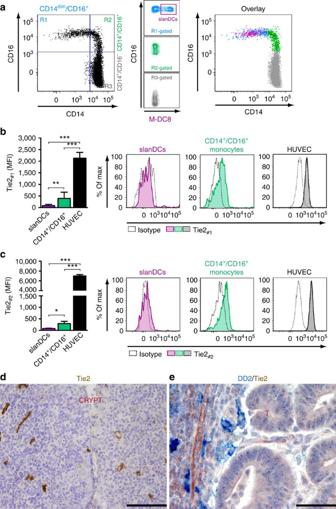Figure 7: Circulating and tissue slanDCs in tonsils and M-TDLN do not express Tie2. (a) Gating strategy used to identify monocyte subpopulations (on the basis of CD14 and CD16 expression) and slanDCs (on the basis of M-DC8 staining within the CD14dim/CD16+subset) in PBMC. (b,c) HUVEC and slanDCs or CD14+/CD16+monocytes within PBMC were analysed for Tie2 expression by flow cytometry using two different anti-human Tie2 monoclonal antibodies (Tie2#1, a PE anti-Tie2 mouse IgG1 from R&D inb; Tie2#2, a PE anti-Tie2 mouse IgG1 from BioLegend inc). Bar graphs reporting the mean±s.d. (n=5–10) are also shown. ***P<0.001; **P<0.01; *P<0.05, by ANOVA. Representative histograms from five experiments with similar results are shown. (d,e) Sections are from a frozen tonsil (d) and fixed M-TDLN (e), stained as indicated and counterstained with Meyer’s haematoxylin. Tie2 staining with two different antibodies fails to recognize slanDCs in M-TDLN (e), while it is very intense in vessel endothelium (d,e). T, tumour cells. Original magnifications: 200X (d, scale bar, 100 μm) and 400X (e, scale bar, 50 μm). Figure 7: Circulating and tissue slanDCs in tonsils and M-TDLN do not express Tie2. ( a ) Gating strategy used to identify monocyte subpopulations (on the basis of CD14 and CD16 expression) and slanDCs (on the basis of M-DC8 staining within the CD14 dim /CD16 + subset) in PBMC. ( b , c ) HUVEC and slanDCs or CD14 + /CD16 + monocytes within PBMC were analysed for Tie2 expression by flow cytometry using two different anti-human Tie2 monoclonal antibodies (Tie2 #1 , a PE anti-Tie2 mouse IgG1 from R&D in b ; Tie2 #2 , a PE anti-Tie2 mouse IgG1 from BioLegend in c ). Bar graphs reporting the mean±s.d. ( n =5–10) are also shown. *** P <0.001; ** P <0.01; * P <0.05, by ANOVA. Representative histograms from five experiments with similar results are shown. ( d , e ) Sections are from a frozen tonsil ( d ) and fixed M-TDLN ( e ), stained as indicated and counterstained with Meyer’s haematoxylin. Tie2 staining with two different antibodies fails to recognize slanDCs in M-TDLN ( e ), while it is very intense in vessel endothelium ( d , e ). T, tumour cells. Original magnifications: 200X ( d , scale bar, 100 μm) and 400X ( e , scale bar, 50 μm). Full size image slanDCs contact innate and adaptive immune cells in M-TDLN Noteworthy, based on quantification performed on double-stained sections, we found that a variable fraction of slanDCs is in contact either with CD56 + NK cells (10±6.5%, n =5) or CD66b + neutrophils (14±11%) in M-TDLN ( Fig. 8a,b ), consistent with the establishment of a potential functional network among slanDCs, neutrophils and NK cells, as previously shown [17] . Most slanDCs (91±4%) regularly interact with CD3 + -T cells, particularly CD4 + -T cells ( Fig. 8c,d ). As quantified by capturing identical microscopic areas of digitalized slides obtained from serial sections of M-TDLN ( Supplementary Fig. S7 ), T lymphocytes in slanDC-rich areas included a significantly dominant GATA3 + population admixed to more rare T-Bet + and Foxp3 + regulatory T cells ( Fig. 8e ; Supplementary Table S3 ). A similar pattern was observed in the group of M-TDLN lacking slanDCs ( Fig. 8e ; Supplementary Table S3 ), indicating that a Th2-type immune response regularly prevails in M-TDLN. Altogether, these findings indicate that, in advanced stage cancer (for example, with nodal spread), slanDCs interact with other immune cells in a dominant Th2-polarized nodal microenvironment. 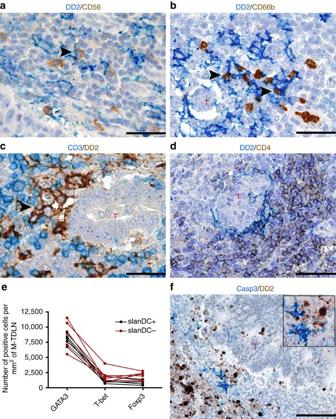Figure 8: slanDCs interactions in Th2-polarized M-TDLN. (a–d) Double staining of sections from representative M-TDLN cases (n=5) show that slanDCs are in contact with CD56+NK cells (a, arrow head), CD66b+neutrophils (b, arrow heads) and CD3+T cells (c, arrow head), the latter population mainly represented by CD4+T cells (d). Graph in (e) illustrates the quantitative analysis of cells expressing GATA3, T-Bet and Foxp3 in M-TDLN (n=10). (fwith insert) slanDCs in M-TDLN were often found in close proximity to apoptotic cells/bodies as demonstrated by double staining with active caspase 3 (n=5). T, tumour cells. Sections are counterstained with Meyer’s haematoxylin. Original magnifications: 600X (a–c, scale bar, 33 μm); 400X (d, scale bar, 50 μm) and 200X (f, scale bar, 100 μm). Figure 8: slanDCs interactions in Th2-polarized M-TDLN. ( a – d ) Double staining of sections from representative M-TDLN cases ( n =5) show that slanDCs are in contact with CD56 + NK cells ( a , arrow head), CD66b + neutrophils ( b , arrow heads) and CD3 + T cells ( c , arrow head), the latter population mainly represented by CD4 + T cells ( d ). Graph in ( e ) illustrates the quantitative analysis of cells expressing GATA3, T-Bet and Foxp3 in M-TDLN ( n =10). ( f with insert) slanDCs in M-TDLN were often found in close proximity to apoptotic cells/bodies as demonstrated by double staining with active caspase 3 ( n =5). T, tumour cells. Sections are counterstained with Meyer’s haematoxylin. Original magnifications: 600X ( a – c , scale bar, 33 μm); 400X ( d , scale bar, 50 μm) and 200X ( f , scale bar, 100 μm). Full size image slanDCs from CCR patients are functionally competent By screening a set of slanDC + M-TDLN using active caspase 3 staining, we found that cell death is abundant and very common particularly within and around metastatic tumour nests ( Supplementary Fig. S8 ). Significantly, a fraction of M-TDLN-associated slanDCs (16±9%, n =5) was found in close proximity to apoptotic cells/bodies, as revealed on double staining for active caspase 3 and DD2 ( Fig. 8f ; insert). Thereby, we tested whether slanDCs could phagocytose apoptotic tumour cells in vitro . To this end, we co-incubated freshly isolated slanDCs with apoptotic cells previously prepared from a panel of colon carcinoma cell lines, namely HT29 and SW480 cells from primary tumours, and SW620 and LOVO cells from metastatic lymph nodes. As shown in Fig. 9a , slanDCs variably, but very efficiently, phagocytosed tumour cell-derived apoptotic bodies, displaying similar or -for SW480 cell line- significantly higher phagocytic capacity than CD1c + DCs from the same healthy donors. Under these experimental conditions, CD14 + monocytes and pDCs displayed, respectively, the highest and the lowest phagocytosing capacity ( Fig. 9a ). We also observed that the uptake of tumour-cell-derived apoptotic bodies by slanDCs is Dectin-1/CLEC7A- and CD18-independent, and that IFNγ- activated slanDCs cultured with fluorescent-labelled, alive HT29 cells contained intracellular apoptotic bodies likely derived from the slanDC-mediated killing of HT29 cells, as previously shown [16] . 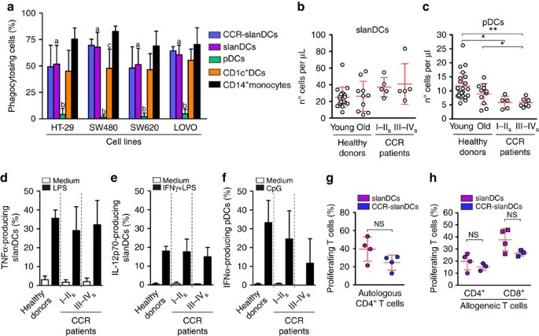Figure 9: Circulating slanDCs from CCR patients remain intact in terms of number and functional properties. (a) CCR-derived slanDCs and healthy donor-derived slanDCs, CD1c+DCs, pDCs, CD14+monocytes were co-incubated for 18 h with apoptotic bodies derived from the indicated colon adenocarcinoma cell lines at 1:3 ratio. Graph shows the net phagocytosis by each cell type calculated as it follows: % of phagocytosing cells at 37 °C—% of phagocytosing cells at 4 °C (mean±s.d.;n=4). Statistical significance, by one-way ANOVA, is also indicated:aversusb,P<0.001;aversusc,P<0.05. (b,c) Quantification of circulating pDCs and slanDCs (mean±s.d.) in young (n=18–23; age mean=37; age range=22–51) and old (n=10–11; age mean=76; age range=68–86) healthy donors, as well as CCR-bearing patients (n=10–12; age mean=73; age range=53–86), further divided into two groups according to their staging (I-IIs=stages I and II; III-IVs=stages III and IV). Symbols stand for: **P<0.01; *P<0.05, by Student’st-test of unpaired samples. (d–f) Graphs show the percentage (mean±s.d.) of TNFα- (d,n=4–7), IL-12p70- (e,n=3–4) producing slanDCs and IFNα-producing pDCs (f,n=3–4) by resting and stimulated PBMC from healthy donors or CCR-bearing patients. % of cytokine- secreting cells was calculated on live M-DC8+slanDC- or CD303+pDC-gated cells. (g,h) Graphs report the percentage of proliferating autologous CD4+T cells (g) or allogeneic CD4+or CD8+T cells (h) cultured for 7 days with healthy donor- or CCR patient-derived slanDCs in the presence (g) or the absence (h) of tetanus toxoid (mean±s.d.;n=3–4). Figure 9: Circulating slanDCs from CCR patients remain intact in terms of number and functional properties. ( a ) CCR-derived slanDCs and healthy donor-derived slanDCs, CD1c + DCs, pDCs, CD14 + monocytes were co-incubated for 18 h with apoptotic bodies derived from the indicated colon adenocarcinoma cell lines at 1:3 ratio. Graph shows the net phagocytosis by each cell type calculated as it follows: % of phagocytosing cells at 37 °C—% of phagocytosing cells at 4 °C (mean±s.d. ; n =4). Statistical significance, by one-way ANOVA, is also indicated: a versus b , P <0.001; a versus c , P <0.05. ( b , c ) Quantification of circulating pDCs and slanDCs (mean±s.d.) in young ( n =18–23; age mean=37; age range=22–51) and old ( n =10–11; age mean=76; age range=68–86) healthy donors, as well as CCR-bearing patients ( n =10–12; age mean=73; age range=53–86), further divided into two groups according to their staging (I-IIs=stages I and II; III-IV s =stages III and IV). Symbols stand for: ** P <0.01; * P <0.05, by Student’s t -test of unpaired samples. ( d – f ) Graphs show the percentage (mean±s.d.) of TNFα- ( d , n =4–7), IL-12p70- ( e , n =3–4) producing slanDCs and IFNα-producing pDCs ( f , n =3–4) by resting and stimulated PBMC from healthy donors or CCR-bearing patients. % of cytokine- secreting cells was calculated on live M-DC8 + slanDC- or CD303 + pDC-gated cells. ( g , h ) Graphs report the percentage of proliferating autologous CD4 + T cells ( g ) or allogeneic CD4 + or CD8 + T cells ( h ) cultured for 7 days with healthy donor- or CCR patient-derived slanDCs in the presence ( g ) or the absence ( h ) of tetanus toxoid (mean±s.d. ; n =3–4). Full size image Circulating mDCs and pDCs from cancer patients are frequently reduced in number and functionally defective [30] , [31] , [32] , [33] , [34] . Recent works have proved the prognostic significance of the immune response to colon carcinomas (CCR) [35] , [36] . By testing a cohort of CCR patients (details are reported in Supplementary Table S4 ), we found that the absolute number of peripheral slanDCs trended towards an increase as compared with those of both younger- or age-matched healthy donors ( Fig. 9b ). By contrast, pDCs from the same patient cohort were significantly reduced in number, not only in an age-dependent but also in a cancer-related manner ( Fig. 9c ), in line with published observations [31] , [34] , [37] , [38] , [39] . Concomitantly, we also found that either the ability to ingest tumour cell-derived apoptotic bodies ( Fig. 9a ), or the capacity to produce and release TNFα and IL-12p70 in response to, respectively, lipopolysaccharide (LPS) and LPS plus IFNγ ( Fig. 9d,e ), was fully retained by CCR slanDCs. By contrast, the capacity of CCR-derived pDCs to produce IFNα upon CpG stimulation was partially defective ( Fig. 9f ), as largely documented in patients with other carcinoma types [34] , [40] , [41] . Significantly, number and function (for example, cytokine production) of the slanDC contingent was maintained even in advanced disease stages ( Fig. 9b,d,e ). Moreover, slanDCs from CCR patients retained the ability to stimulate T-cell proliferation in both autologous ( Fig. 9g ) and allogeneic settings ( Fig. 9h ). Supernatants harvested from colon carcinoma metastatic cell lines (such as SW620, LOVO and COLO-678) influenced neither the capacity of IFNγ plus LPS-activated slanDCs to produce TNFα or IL-12p70, nor their survival rate ( Supplementary Fig. S9 ). Finally, to identify potential mediators responsible for slanDC migration to M-TDLN, we initially tested the expression levels of a set of chemotactic receptors by slanDCs. As a result, we uncovered that slanDCs from CCR subjects displayed slightly higher, but not statistically significant, levels of surface CXCR4 than control slanDCs, in contrast to surface CX3CR1 and C5aR, which were expressed at identical amounts on the two slanDC populations ( Fig. 10a,b ). As expected [14] , CCR2, CCR3, CCR5 and CXCR3 were expressed neither in slanDCs from healthy donors nor in slanDCs from CCR subjects. Importantly, chemotaxis induced by CXCR4, CX3CR1 or C5aR ligands was substantially equivalent in slanDCs derived from CCR subjects and healthy controls ( Fig. 10c ). These findings are relevant, as the ligands for CXCR4, CX3CR1 and C5aR, respectively CXCL12/SDF-1, CX3CL1/Fractalkine and C5a, are strongly expressed in M-TDLN where slanDCs are found ( Fig. 10d–i ). Specifically, CXCL12/SDF-1 and CX3CL1/Fractalkine were detected primarily in tumour cells, nodal stromal cells and, particularly in the case of CXCL12/SDF-1, in the HEV endothelium. In contrast, C5a was detected in nodal macrophages and other CD11c + cells ( Fig. 10f ; insert). Remarkably, a strong CXCL12/SDF-1 and CX3CL1/Fractalkine signal in M-TDLN was evident also in tumour cells adjacent to slanDCs ( Fig. 10g,h ). However, when tested in TMA, as well as in a set of eight carcinoma cases for which matched PC and M-TDLN were available, we detected similar CXCL12, CX3CL1 and C5a expression levels also in PC. 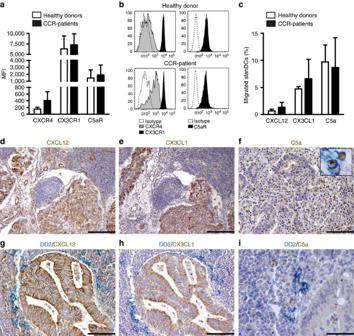Figure 10: Migratory properties by slanDCs from CCR patients and chemokine expression in M-TDLN. (a,b) Freshly isolated PBMC from healthy donors and CCR patients were analysed for C5aR, CXCR4 and CX3CR1 expression on gated M-DC8+slanDCs, by flow cytometry. (a) Data for each chemokine receptor are reported as mean fluorescence intensity (after the subtraction of the mean fluorescence intensity given by the correspondent isotype control antibody, mean±s.d.;n=6). (b) Representative histograms of CXCR4, CX3CR1 and C5aR expression by slanDCs from healthy donors and CCR patients are shown. (c) Graph shows the percentage of migrating slanDCs towards CXCL12, CX3CL1 and C5a in chemotaxis assays (n=4). (d–i) Sections from slanDCs positive M-TDLN representative cases (n=10) stained as indicated. CXCL12/SDF-1 and CX3CL1/Fractalkine are detected in tumour cells, nodal stromal cells and, for CXCL12/SDF-1, also in HEV endothelium (serial sectionsd,eandg,h). C5a is mainly expressed by nodal stromal cells (f,i), some of them expressing CD11c (blue, insert inf). T, tumour cells. Sections are counterstained with Meyer’s haematoxylin. Original magnifications: 100X (d,e, scale bar, 200 μm); 200X (f–h, scale bar, 100 μm) and 400X (i, scale bar, 50 μm). Figure 10: Migratory properties by slanDCs from CCR patients and chemokine expression in M-TDLN. ( a , b ) Freshly isolated PBMC from healthy donors and CCR patients were analysed for C5aR, CXCR4 and CX3CR1 expression on gated M-DC8 + slanDCs, by flow cytometry. ( a ) Data for each chemokine receptor are reported as mean fluorescence intensity (after the subtraction of the mean fluorescence intensity given by the correspondent isotype control antibody, mean±s.d. ; n =6). ( b ) Representative histograms of CXCR4, CX3CR1 and C5aR expression by slanDCs from healthy donors and CCR patients are shown. ( c ) Graph shows the percentage of migrating slanDCs towards CXCL12, CX3CL1 and C5a in chemotaxis assays ( n =4). ( d – i ) Sections from slanDCs positive M-TDLN representative cases ( n =10) stained as indicated. CXCL12/SDF-1 and CX3CL1/Fractalkine are detected in tumour cells, nodal stromal cells and, for CXCL12/SDF-1, also in HEV endothelium (serial sections d , e and g , h ). C5a is mainly expressed by nodal stromal cells ( f , i ), some of them expressing CD11c (blue, insert in f ). T, tumour cells. Sections are counterstained with Meyer’s haematoxylin. Original magnifications: 100X ( d , e , scale bar, 200 μm); 200X ( f – h , scale bar, 100 μm) and 400X ( i , scale bar, 50 μm). Full size image Altogether, these data indicate that the expansion of fully competent circulating slanDCs in CCR patients might significantly contribute to kill and capture tumour cells, efficiently present antigens to T cells and deliver elevated amounts of TNFα and IL-12p70. Our data also imply that C5a, CX3CL1/Fractalkine and CXCL12/SDF-1, which are abundantly produced by carcinoma cells and nodal stromal cells, participate to the specific homing of slanDCs to inflamed M-TDLN. Although slanDCs represent the most abundant CD11c + mDCs in humans [11] , and characteristically display efficient proinflammatory properties [11] , [13] , [15] , their role in cancer immunoediting has never been explored, likely because their murine counterpart has not been identified yet. Therefore, in this study, we made a systematic characterization of slanDCs in human cancers and, as a result, we could identify slanDCs as new players in cancer immunity for their direct participation in the organization of nodal immune responses to transformed epithelial cells. We, in fact, found that slanDCs distinctively home to M-TDLN in patients affected by different forms of carcinomas. Remarkably, slanDCs are absent in PC, while their nodal recruitment follows the arrival of carcinoma cells to M-TDLN, as indicated by the analysis of SLNs from breast cancer patients. The complete absence of slanDCs in the PC microenvironment was confirmed by analysing multiple sections of different PC tumour blocks with their matched M-TDLN, the latter of which contained high numbers of slanDCs. Of note, the majority of PC analysed in this study contained sizeable numbers of macrophages and other DC subtypes. Moreover, based on a series of investigations on their distribution and phenotype in vivo and in vitro , we were able to demonstrate that slanDCs are clearly distinct from TEMs, a subset of CD16 + monocytes that infiltrates PC and were recently described to have pro-angiogenic activities [26] . Finally, slanDCs behave differently compared with other nodal DCs in M-TDLN. In fact, pDCs and iDCs were expanded in number in M-TDLN, but maintained normal localization patterns, whereas slanDCs were selectively juxtaposed with neoplastic nests at interfaces between cancer cells and lymphoid cells. This large set of data establishes the uniqueness of carcinoma-associated slanDCs, and illustrates that they are distinct from other major tumour-associated leukocyte populations. Our data also suggest that slanDC-homing to TDLN represents an early event that specifically requires the co-occurrence of intranodal malignant cell deposits. Prior studies had shown that migration of circulating slanDCs to tissues is guided by a set of chemotactic receptors including CXCR4, CX3CR1 and C5aR [11] , [14] . Accordingly, we found that CXCL12/SDF-1, CX3CL1/fractalkine and C5a, the ligands for these receptors, are abundantly produced in M-TDLN, either by lymph node cells (for example, HEV and stromal cells within the interfollicular areas) or by carcinoma cells. Moreover, by studying a cohort of CCR patients, we also demonstrate that CXCR4, CX3CR1 and C5aR are normally expressed and functional in circulating slanDCs. Noteworthy, CX3CL1/fractalkine is already known to be specifically released by apoptotic cells to attract leukocytes at the site of high-rate cell death [42] , [43] , [44] . However, the fact that we found CXCL12/SDF-1, CX3CL1/fractalkine and C5a expressed also in the PC (that do not contain slanDCs) clearly indicates that recruitment of tumour-associated slanDCs require a complex assembly of cellular and molecular components governed by M-TDLN. We therefore postulate that a specific set of adhesion molecules, likely expressed by HEV of inflamed M-TDLN, might be crucial for the slanDC entry into the node. We envisage that specific mechanisms could be also operative in peripheral tissues of patients with autoimmune diseases, such as Crohn’s disease, rheumatoid arthritis, psoriasis [13] , [14] , [17] and lupus erythematosus [45] , especially when slanDC infiltration is associated to highly dense chronic inflammation, particularly in the form of lymph follicle-like structures [45] . Another novel finding highlighted in this study is the peculiar localization of slanDCs in M-TDLN. We uncovered that slanDCs are frequently poised at the interface between tumour nests and lymphoid compartments, thus allowing a two-way direct interaction with both neoplastic cells and T cells. Although presentation of tumour antigens by activated DCs is retained in TDLN, most phagocytosis of tumour-derived antigens is exerted by immature DCs in the PC. Prompted by the observations that slanDCs display a phagocytic morphology (for example, large cytoplasm containing intracellular debris), and contact apoptotic caspase 3 + cells within metastatic nests, we analysed their ability to phagocytose tumour cells in vitro . By using a panel of tumour cell lines, we demonstrated that slanDCs displayed a similar or—for some cell lines—a greater phagocytic capacity than classical CD1c + DCs from the same donor. Thus, the observed features of slanDCs in M-TDLN (for example, localization close to metastatic cells and phagocytic capacity) are of remarkable biological and clinical relevance, as these findings imply that tumour antigens derived from carcinoma cells in M-TDLN could be directly presented to T cells by nearby slanDCs. This hypothesis is consistent with recent observations, made by intravital live imaging, clarifying that CD11c + DCs poised at the tumour margin constitutively ingest tumour-derived proteins and present processed tumour antigens to reactive T cells [46] . In addition, slanDC interactions with either NK cells or neutrophils occurring in M-TDLN might further amplify nodal immune responses, thus extending our previous observations on the presence of slanDC/neutrophil/NK cell networks in inflamed mucosal tissues [17] . Remarkable results have been recently obtained by analysing the significance of the ‘immune contexture’ of primary tumours in large cohorts of clinical samples [47] ; however, it still remains difficult to establish the specific contribution of the innate immune cell compartment to cancer immunity. In M-TDLN, although we could detect some levels of activation of slanDCs (by measuring TNFα and co-stimulatory molecule expression), the analysis of nodal T-cell compartment showed a dominant Th2-type polarization irrespective of the slanDC content. This might reflect the prevalence of an immune suppressive environment in advanced stage of cancer (for example, carcinomas with nodal metastasis). Whatever the case is, circulating slanDCs obtained from healthy donors, cultured in carcinoma cell-conditioned medium, remain fully competent in terms of TNFα and IL-12p70 production, and do not display an altered viability. More importantly, by analysing circulating slanDCs from a cohort of patients with advanced CCR, we found that the slanDC compartment, unlike pDCs from the same patient cohort, remains substantially intact in terms of number and responsive to stimuli in terms of cytokine (TNFα and IL-12p70) production, induction of T-cell proliferation as well as gene expression profile by microarray analysis, even in advanced stage disease. Thus, in contrast to other DC subsets [7] , [34] , our data suggest that circulating slanDCs are not developmentally or functionally hijacked by growing tumours and converted into immunosuppressive cells. If so, we would further propose that, in advanced stage carcinoma, when other circulating DCs are dysfunctional [4] , [6] , [7] , [8] and migration to draining lymph nodes is impaired [48] , or the source of tumour antigens in the PC has been surgically removed, circulating slanDCs might still represent a highly qualified second line defence to be exploited. Tissues FFPE tissue blocks used for this study were retrieved from the tissue bank of the Department of Pathology (Spedali Civili di Brescia, Brescia, Italy). Human tissues included normal thymus, spleen and bone marrow, reactive lymphoid organs (tonsils, lymph nodes, appendix) as well as normal non-lymphoid tissues (ileum, colon, stomach, oesophagus, thyroid, salivary gland, oral mucosa, breast, lung, brain, liver, pancreas, skin, kidney, ureter, bladder, testis, prostate, ovary, endometrium, cervix). Pathological samples used for slanDC analysis included multi-tumour TMA of mixed carcinomas (( Supplementary Table S1 ), see below for technical details), sections of 10 primary cutaneous melanoma cases, 80 metastatic tumour-draining lymph nodes (M-TDLN) (details are in Supplementary Table S2 ), 155 non-metastatic tumour-draining lymph nodes (non-metastatic TDLN), from cutaneous melanoma, head and neck squamous cell carcinoma and colon carcinoma, respectively, and a cohort of 52 distant metastasis to different organs (liver, lung, brain, omentum, small intestine) derived from a set of PCs from different sites (urinary tract, GI tract, breast, ovary, lung, head and neck and skin). For a subgroup of 14 M-TDLN, the matched primary tumour samples were also available (allowing comparative analysis). An additional group of TDLN included 51 metastatic SLNs (M-SLNs) and 22 NM-SLNs from breast cancer patients. Finally, 13 lymph nodes containing benign salivary gland epithelial inclusions were also analysed. Tissue microarray preparation Three tissue microarray (TMA) blocks were prepared from a series of 126 PCs from different sites, as detailed in Supplementary Table S1 . TMAs were constructed using an automated tissue microarrayer (TMA Master, 3DHistech). Three representative tumour areas were identified on haematoxylin and eosin (H&E)-stained sections. For each area, a 1 mm core was obtained by punching the original tissue block. Four-micron thick tissue sections were H&E stained and checked for tumour cell content. Sections and stainings on TMA were performed as described below. For scoring and panel preparation, stained sections were digitalized by using the Aperio Scanscope System. Digital Images were taken as snapshots by using Imagescope software and resized by using Adobe Photoshop. Immunohistochemistry and immunofluorescence Four-micron thick tissue sections were used for immunohistochemical staining. slanDCs were identified by using primary antibodies towards 6-sulfo LacNAc residue (slan/M-DC8) on PSGL-1, namely clones DD1 and DD2, as previously reported [13] . The reaction was revealed using Novolink Polymer (Leica Microsystems) followed by DAB. For double immunohistochemistry, DD2 was coupled with a panel of markers ( Supplementary Table S5 ). Briefly, after completing the first immune reaction, the second was visualized using Mach 4 MR-AP (Biocare Medical), followed by Ferangi Blue (Biocare Medical) as chromogen. For immunofluorescence, DD1 or DD2 were used in combination with CD11c, CD68, S100 protein and CD3 (see Supplementary Table S5 for detection system and antibody dilutions), and then sections were counterstained with 4',6-diamidino-2-phenylindole. slanDC interactions were analysed by capturing at least three high power fields/M-TDLN, on double-stained sections. The Th-type polarization was defined by automatic cell counting of positive cells on digitalized slides (Aperio Scanscope, IHC Nuclear algorithm) obtained from serial sections immunostained, respectively, for GATA3, T-Bet and Foxp3. Selection of the T-cell area in slanDC-containing M-TDLN was based on the occurrence of slanDCs, as proved by DD1 stain on serial sections. All isotype control stains are reported in Supplementary Fig. S10 . Cell isolation and culture PBMC were isolated under endotoxin-free conditions [49] from the whole blood of healthy donors and 22 patients bearing colon adenocarcinoma (see Supplementary Table S4 for clinical details). slanDCs, CD1c + DCs, pDCs and CD14 + monocytes were isolated either from buffy coats of healthy donors and/or from the blood of CCR patients using specific isolation kits from Miltenyi Biotec, according to the manufacturer’s instructions. In the case of CD4 + T or pan T lymphocytes, cells were isolated from PBMC using, respectively, the EasySep Human CD4 + T Cell Enrichment Kit (StemCell Technologies) and the Human Pan T Cell Isolation Kit II (Miltenyi Biotec, Bergisch Gladbach, Germany). After isolation, cells were suspended in standard medium (RPMI 1640 medium supplemented with 10% low-endotoxin fetal bovine serum (<0.5 endotoxin units ml −1 Lonza, Basel, Switzerland)) and were either immediately analysed after isolation for antigen expression or cultured up to 18 h in 48-/96-well tissue culture plates for functional assays (see below). Tonsils, obtained from patients affected by hypertrophic tonsils or recurrent, chronic tonsillitis and thus undergoing surgery via cold steel dissection, were minced into small fragments, treated for 15 min at 37 °C with 0.2 mg ml −1 Liberase Blendzyme 2 (Roche, Basel, Switzerland), and processed by gentleMACS dissociator (Miltenyi Biotec), according to the manufacturer’s instructions. Tonsil cell suspensions were then washed, filtered through a 40 μm cell strainer and enriched in DCs fraction by depleting T and B lymphocytes with CD3 and CD19 MicroBeads (Miltenyi Biotec). All experimental procedures were approved by the institutional review boards of the University of Verona and Spedali Civili of Brescia. All human samples were obtained following patients’ informed written consent. Cell lines Five (mycoplasma-negative) human colon adenocarcinoma cell lines were used in this study, namely the SW480-primary and SW620-matched lymph node metastatic cell lines (from ICLC, National Institute for Cancer Research, Genoa, Italy), the COLO-678-metastatic cell line (from DSMZ, Braunschweig, Germany), the HT-29-primary and the LOVO-lymph node metastatic cell lines (kindly provided by Dr Claudio Sorio, Department of Pathology and Diagnostics, University of Verona, Italy). Cell lines were cultured in Dulbecco's Modified Eagle Medium supplemented with 10% FBS, with the exception of SW480 cells (cultured in standard medium). Human umbilical vein endothelial cells were grown on fibronectin-coated flasks using the EGM-2 Bullet Kit (Lonza). Flow cytometry For phenotypic studies by flow cytometry, usually 250,000 PBMC or 100,000 cells from tonsil suspensions were first incubated for 5 min in 50 μl PBS containing 5% human serum (to prevent nonspecific binding), and then stained for 15 min at room T using the monoclonal antibodies listed in Supplementary Table S6 , which also specifies their working dilution. Sample fluorescence was measured by a seven-colour MACSQuant Analyzer (Miltenyi) or a six-colour FACSCanto II (BD Biosciences, Franklin Lakes, NJ). Data analysis was performed by FlowJo software Version 8.8.6 (TreeStar). Phenotypic cell analysis under the various experimental conditions was performed in live cells, identified as either Vybrant DyeCycle Violet- or propidium iodide-negative cells (Life Technologies, Carlsbad, CA). Count of peripheral blood DCs To count the absolute number of circulating slanDCs and pDCs, 50 μl of whole blood from healthy donors and cancer-bearing patients were stained for 15 min at room T with brilliant violet 510 anti-human CD45, APC-Cy7 anti-human HLA-DR, PE-Cy7 anti-human CD56/CD3/CD19 (LIN), PerCP-Cy5.5 anti-human CD16, PE anti-human CD123 and FITC anti-human CD303 or M-DC8 mAbs, at the working dilution specified in Supplementary Table S6 . Samples were then incubated for 10 min with RBC Lysis Solution (Qiagen, Venlo, Limburg, Netherlands), washed and analysed by MACSQuant Analyzer (Miltenyi Biotec). slanDCs and pDCs were identified, respectively, as HLA-DR + /CD16 + /M-DC8 + and HLA-DR + /CD123 + /CD303 + cells within the CD45 + /LIN − cells. The absolute number of DCs per μl was calculated by multiplying the hemocytometer white blood cell count (performed independently on whole-blood samples) to the DC percentage among the CD45 hi -gated cells. Analysis of cytokine production PBMC were tested for IL-12p70, TNFα and IFNα production by specific cytokine secretion assays (Miltenyi Biotec) [17] . Briefly, 500,000 PBMC isolated from both healthy donors and colorectal cancer-bearing patients were incubated with 100 ng ml −1 LPS (Ultra-Pure E. coli LPS (0111:B4 strain) from Alexis Biochemicals, San Diego, CA) for 4 h at 37 °C in standard medium to optimally detect TNFα. Alternatively, PBMC were first cultured for 6 h and then stimulated for additional 12 h with either 100 ng ml −1 LPS plus 100 U ml −1 IFNγ (R&D Systems), or 5 μg ml −1 CpG oligonucleotides type A (ODN-2216 from InvivoGen, San Diego, CA), to optimally detect IL-12p70 and IFNα, respectively. slanDC- or pDC-producing cytokines were identified by MDC-8- or CD303-positivity, once analysed by MACSQuant Analyzer (Miltenyi Biotec). Immunoblots Whole-cell extracts prepared from both freshly isolated slanDCs and human umbilical vein endothelial cells by the RNeasy mini kit (Qiagen) [50] were processed for immunoblotting using two different anti-Tie2 Abs (C-20, a mAb from Santa Cruz Biotechnology, at 1:200 dilution and 0.2 μg ml −1 goat polyclonal Ab from R&D Systems). An anti-β-actin mAb (Sigma, St Louis, Missouri, at 1:2,000 dilution) was also used to check for equal protein loading. Blotted proteins were quantified by Odyssey infrared imaging system (LI-COR Biosciences, Lincoln, Nebraska). Quantitative RT–PCR Real time quantitative polymerase chain reaction was performed as described [51] using the following primer pairs (Invitrogen): forward 5′-CTGTTAAAGTTCTTCCAAAGCC-3′ and reverse 5′-CATATTCTGTCCGAGGTTCCA-3′ for Tie2; forward 5′-AGGGTTCGTAGAAGATTCAAGG-3′ and reverse 5′-GGAAACATTGTGAGCGATCTC-3′ for RPL32. Data were calculated by Q-Gene software ( http://www.gene-quantification.de/download.html#qgene ) and expressed as mean normalized expression units after RPL32 normalization. Chemotaxis assay Chemotactic assays were performed as described by Hansel et al. [14] , with minor modifications. Briefly, 75 μl of PBMC suspensions (7 × 10 6 cells per ml) in RPMI medium containing 10% FBS were seeded into the upper transwell inserts (5-μm pore filter) of a 96-well chemotaxis chamber. 10 ng ml −1 C5a, CXCL12/SDF-1 (R&D Systems) or CX3CL1/Fractalkine (Peprotech, Rocky Hill, NJ) were added to the bottom wells and, after 1.5 h, transmigrated cells were stained with CD16 and M- DC8 mAbs (for slanDC identification) and quantified by flow cytometry. Migration is given as migrated slanDCs, calculated as percentages of input (slanDCs initially present in the PBMC cell suspension). Apoptotic cell uptake assay Purified slanDCs, CD1c + DCs, pDCs and CD14 + monocytes were plated for 18 h in U-bottom 96-well plates in the presence of apoptotic bodies previously prepared from tumour cell lines, as follows. Tumour cell lines were cultured under adherent conditions in 24-well plates and, once confluent, labelled with 5 μM CellTracker Green CMFDA (Molecular Probes). Cells were then washed, irradiated and cultured under serum-free conditions. After 24 h, non-adherent dead cells were collected (being, on average, 45% apoptotic and 55% necrotic, as assessed by Violet Chromatin Condensation/Dead Cell Apoptosis Kit (Invitrogen)), washed, counted and finally added to 2.5 × 10 4 slanDCs from healthy donors or CCR patients, or to CD1c + DCs, pDCs and CD14 + monocytes from healthy donors at a 1/1-1/3 ratio (DCs/dead cells) for 15 h at both 37 °C and at 4 °C. The latter condition was used to determine the basal % of phagocytosing DCs/monocytes (always≤5%). Plates were then centrifuged at 300 × g for 10 min, medium removed and cells suspended in HBSS buffer containing 1 μM VybrantTM DyeCycleTM Violet stain (Molecular Probes, Eugene, Oregon) and HLA-DR APC- Cy7 for 30 min on ice. Phagocytosing cells were defined, by flow cytometry, as those cells that resulted CMFDA green fluorescence-positive among the Vybrant − /HLA-DR + cells (live DCs/monocytes). T-cell proliferation assay Freshly isolated slanDCs (5 × 10 3 ) from both healthy donors and CCR patients were co-cultured either with 5 × 10 4 CFSE-labelled autologous CD4 + T lymphocytes, in the absence or presence of 5 μg ml −1 tetanus toxoid [15] , or with 5 × 10 4 CFSE-labelled allogeneic pan T lymphocytes in U-bottomed 96-well plates (Costar, Corning Incorporated, Corning, NY). Under the latter experimental conditions, CD4 + and CD8 + T-cell populations were identified, respectively, as CD3 + /CD4 + and CD3 + /CD8 + cells, by flow cytometry. T-cell proliferation was assessed by CFSE dilution on day 7. Statistical analysis Data are expressed as mean±s.d. of the number of experiments indicated in each figure legend. Statistical analysis, including two-tailed Student’s t -test, Fisher test, one-way or two-way analysis of variance was performed by Prism Version 4.0 software (GraphPad). How to cite this article : Vermi, W. et al. slanDCs selectively accumulate in carcinoma-draining lymph nodes and marginate metastatic cells. Nat. Commun. 5:3029 doi: 10.1038/ncomms4029 (2014).